Dietary methionine can sustain cytosolic redox homeostasis in the mouse liver Across phyla, reduced nicotinamide adenine dinucleotide phosphate (NADPH) transfers intracellular reducing power to thioredoxin reductase-1 (TrxR1) and glutathione reductase (GR), thereby supporting fundamental housekeeping and antioxidant pathways. Here we show that a third, NADPH-independent pathway can bypass the need for TrxR1 and GR in mammalian liver. Most mice genetically engineered to lack both TrxR1 and GR in all hepatocytes (‘TR/GR-null livers’) remain long-term viable. TR/GR-null livers cannot reduce oxidized glutathione disulfide using NADPH but still require continuous glutathione synthesis. Inhibition of cystathionine γ-lyase causes rapid necrosis of TR/GR-null livers, indicating that methionine-fueled trans -sulfuration supplies the necessary cysteine precursor for glutathione synthesis via an NADPH-independent pathway. We further show that dietary methionine provides the cytosolic disulfide-reducing power and all sulfur amino acids in TR/GR-null livers. Although NADPH is generally considered an essential reducing currency, these results indicate that hepatocytes can adequately sustain cytosolic redox homeostasis pathways using either NADPH or methionine. Aerobic metabolism exposes cellular macromolecules to oxidation. To maintain redox homeostasis, most species, including all vertebrates, have two major cytosolic nicotinamide adenine dinucleotide phosphate- (NADPH) dependent disulfide reductase systems: the thioredoxin (Trx) system and the glutathione (GSH) system [1] , [2] . In mammals, NADPH is generated by glucose oxidation via the pentose phosphate pathway or by other oxidases [3] , [4] , [5] . Critical homeostasis and cytoprotective reactions that require reducing power from the Trx or GSH systems include the synthesis of DNA precursors by ribonucleotide reductase, reduction of cystine into cysteine, reduction of protein disulfides and detoxification of reactive oxygen species [2] , [6] , [7] , [8] , [9] , [10] . GSH is a 307-Da tripeptide ( L -γ-glutamyl- L -cysteinylglycine) that carries reducing power as a transferrable electron on the thiol (-SH) of the cysteine side chain [11] . Typically, two GSH molecules oxidize to form glutathione disulfide (GSSG) in reactions that transfer two electrons of reducing power to an acceptor. GSH reductase (GR) uses electrons from NADPH to reduce the disulfide bond in GSSG, thereby restoring two molecules of GSH [11] . Mice constitutively lacking GR are robustly viable [12] . In addition, although mice constitutively deficient in GSH biosynthesis are embryonic lethal [13] , the reasons for lethality are unclear, as mouse cells unable to synthesize GSH are viable in culture [13] , [14] and organisms of many phyla, including mice, tolerate systemic depletion of GSH [15] , [16] . Cell or organismal survival in the absence of key components of the GSH system is generally explained by redundancies between the GSH and Trx systems. Trxs are small proteins (~12 kDa) that carry two transferrable electrons on an active site cysteine pair via a reversible disulfide/dithiol motif. The disulfide can be recycled to a dithiol by Trx-reductase (TrxR), thereby oxidizing one molecule of NADPH [17] . In mammals, the cytosolic Trx system consists of Trx1 and TrxR1. Trx1-null or TrxR1-null zygotes proliferate to contain several thousand viable cells, but they are disorganized and fail to gastrulate [18] , [19] . Systemic pharmacologic inhibition of TrxR activity in mice or humans is well tolerated [17] and, using conditional alleles to bypass embryonic lethality, it has been shown that TrxR1-null cells and tissues are robust [18] , [20] , [21] . TrxR1-null mouse livers require sustained GSH levels to replicate DNA, suggesting that in the absence of TrxR1, GSH must provide electrons, via glutaredoxin, to ribonucleotide reductase for synthesis of DNA precursors [10] , [22] . This further demonstrates a functional redundancy between the Trx1 and GSH systems that allows survival when either one of the systems is compromised. Although concomitant elimination of both TrxR1 and GSH in hepatocytes blocks DNA replication [10] , it has remained uncertain whether reducing power transferred from intracellular oxidative pathways via NADPH to the cytosolic disulfide reductase systems is an absolute requirement. Interestingly, mutations compromising NADPH production in humans or mice are often non-lethal, although compensatory pathways remain only partially understood [4] , [5] . In the current study, to test whether having at least one of the two major cytosolic NADPH-dependent disulfide reductases is essential for hepatocyte survival in vivo , we ablated Txnrd1 , encoding TrxR1, in the hepatocytes of mice having a germline disruption of Gsr , encoding GR. We show that mice lacking both TrxR1 and GR in all hepatocytes (‘TR/GR-null’ livers) can sustain hepatic redox homeostasis and organismal survival, using the essential amino acid methionine as the liver’s sole detectable source of both cytosolic disulfide-reducing power and sulfur amino acids. This is the first demonstration that an extracellular nutrient, methionine, can supplant the need for intracellular use of NADPH by GR or TrxR1 and sustain cytosolic redox homeostasis in mammalian cells. This study reveals new insights into the diverse mechanisms that cells can use to maintain redox homeostasis, which may be important during acute oxidative challenge as well as support of basal redox processes. TR/GR-null livers require de novo GSH synthesis for survival Initial experiments using fluorescently marked mosaic livers revealed that TR/GR-null hepatocytes are stably persistent in mouse livers, and that adult mice could survive following induced conversion of all hepatocytes to TR/GR null ( Fig. 1 ). Therefore, we generated mice being constitutively whole-liver TR/GR null ( Fig. 2 ). Despite having neither GR nor TrxR1 in any hepatocytes, these mice exhibited no lethality before postnatal day 32 (P32). In most cases, liver histology of post-weaning juveniles (P21–P32) was grossly normal ( Fig. 2a–d ), although some animals exhibited possible oval cell expansions ( Fig. 2d , white arrow) or small necrotic or leukocytic foci ( Fig. 2e , green or yellow arrows, respectively). In animals over 50 days of age, liver histology usually showed leukocytic foci and biliary hyperplasia ( Fig. 2f , yellow and black arrows, respectively), suggesting they were surviving under a state of chronic low-grade hepatic inflammation. Between P32 and P42, mice with TR/GR-null livers exhibited 15% spontaneous lethality, which was associated with global liver necrosis; however, almost no lethality occurred thereafter ( Fig. 2g ). Adult mice with TR/GR-null livers were fertile in both genders, although females were somewhat less fecund than controls (70% litter size, Fig. 2h ). Liver mass in adults was 2.1-fold greater than controls ( Fig. 2i ). Immunoblots on liver samples verified that TR/GR-null livers had almost no TrxR1 protein but normal levels of Trx1 ( Fig. 3a ). Residual TrxR1 in the tissue lysate is likely derived from non-hepatocyte cell types such as endothelia, as shown previously with conditional TrxR1-knockout livers [10] , [20] , [23] . TR/GR-null liver lysates also had no detectable NADPH-dependent GSSG reduction activity ( Fig. 3b ), verifying there was not an alternative NADPH-dependent GSSG reductase supporting homeostasis. TR/GR-null livers had normal concentrations of total GSH and, surprisingly, most of this was in the reduced (GSH) form ( Fig. 3c ). By contrast, total proteins from TR/GR-null livers contained only 85% as many reactive thiols as did those from wild-type livers, suggesting that proteins were more oxidized in the TR/GR-null livers ( Fig. 3d ). During post-hepatectomy regeneration, hepatocyte S-phase indexes were similar in wild-type and TR/GR-null livers ( Fig. 3e ). However, buthionine sulfoximine (BSO), which blocks GSH synthesis, inhibited hepatocyte DNA replication in TR/GR-null livers but not in control livers ( Fig. 3e ). 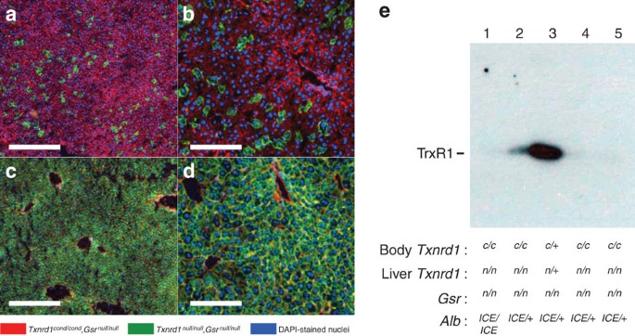Figure 1: Long-term persistence of TR/GR-null hepatocytesin situ. (a,b) Fluorescently marked mosaic analysis of TR/GR-null hepatocyte longevity. An arbitrary subset of hepatocytes in adult ROSAmT-mG/mT-mG;Txnrd1cond/cond;Gsrnull/nullmice were exposed to Cre recombinase by hydrodynamic delivery of plasmid pCMVpCreSVtx, harvested 22 days later and stained with DAPI (4',6-diamidino-2-phenylindole). (c,d) Survival of livers in which most or all hepatocytes are TR/GR-null. Adult ROSAmT-mG/mT-mG;Txnrd1cond/cond;Gsrnull/null; AlbICE/+mice, having Cre expression driven by the AlbICEallele received a single intraperitoneal dose of Tamoxifen. Images shown are DAPI-stained cryosections of livers from mice harvested 4 weeks after Tamoxifen administration. Scale bars, 200 μm (a,c) or 50 μm (b,d). (e) Immunoblots of TrxR1 protein in livers. Mice received a single dose of Tamoxifen as incanddabove and were harvested ≥16 days later. Each lane contained 75 μg of whole liver lysate. Genotypes of the mouse body and liver are indicated below. Residual TrxR1 protein in lane 2 is due either to incomplete conversion or spill-over from lane 3. c, conditional-null allele; n, null allele; +, wild-type allele; ICE, IRES-CreERT2 allele. Figure 1: Long-term persistence of TR/GR-null hepatocytes in situ. ( a , b ) Fluorescently marked mosaic analysis of TR/GR-null hepatocyte longevity. An arbitrary subset of hepatocytes in adult ROSA mT-mG/mT-mG ;Txnrd1 cond/cond ;Gsr null/null mice were exposed to Cre recombinase by hydrodynamic delivery of plasmid pCMVpCreSVtx, harvested 22 days later and stained with DAPI (4',6-diamidino-2-phenylindole). ( c , d ) Survival of livers in which most or all hepatocytes are TR/GR-null. Adult ROSA mT-mG/mT-mG ;Txnrd1 cond/cond ;Gsr null/null ; Alb ICE/+ mice, having Cre expression driven by the Alb ICE allele received a single intraperitoneal dose of Tamoxifen. Images shown are DAPI-stained cryosections of livers from mice harvested 4 weeks after Tamoxifen administration. Scale bars, 200 μm ( a , c ) or 50 μm ( b , d ). ( e ) Immunoblots of TrxR1 protein in livers. Mice received a single dose of Tamoxifen as in c and d above and were harvested ≥16 days later. Each lane contained 75 μg of whole liver lysate. Genotypes of the mouse body and liver are indicated below. Residual TrxR1 protein in lane 2 is due either to incomplete conversion or spill-over from lane 3. c, conditional-null allele; n, null allele; +, wild-type allele; ICE, IRES-CreERT2 allele. 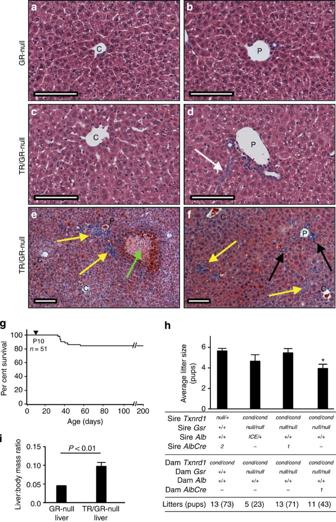Figure 2: Survival and physiological characteristics of mice with TR/GR-null livers. (a–f) Histopathology. As indicated at left, control GR-null livers (a,b) or AlbCre-driven TR/GR-null livers (c–f) are shown from P22 (a–e) or P56 (f) mice. Higher magnification images show representative centrolobular (a,c) or periportal (b,d) regions. White arrow, tract of apparent oval cells; yellow arrows, leukocytic foci; green arrow, necrotic focus, black arrow, biliary expansion. C, central veins; P, portal triad. Scale bars, 100 μm on all panels. (g) Survival of mice with AlbCre-driven TR/GR-null livers. Fifty-one pups from 20 litters with AlbCre-driven TR/GR-null livers were followed. No mice were lost before P32. Between P32 and P42, 15% of the mice were lost. Only one additional loss occurred thereafter (at P55). (h) Gender-specific fecundity. Genotypes of sires and dams for each of four mating classes, as well as the number of litters produced and the pups weaned, are indicated at bottom. For a control (first bar from left), production for the TR-null liver colony was monitored over 13 litters (73 pups), giving an average of 5.6 pups/litter. Fecundity was similar in the mice in which AlbICEdrives conversion of livers to TR/GR-null (4.6 pups/litter, second bar from left). Fecundity was also similar in matings where the sires had AlbCre-driven TR/GR-null livers and the dams had GR-null livers (third bar from left, 5.5 pups/litter). However, when dams with TR/GR-null livers were mated with sires with GR-null livers, production was only 70% (fourth bar from left, 3.9 pups/liter), which was significantly less than the controls (*,P<0.01). None of the first three conditions differed significantly from each other. The five oldest production breeders with TR/GR-null livers in the colony, as of this writing, are all over 365 days old (two female and three male) and in combination have weaned ~30 litters. (i) Adult (P49–64) TR/GR-null liver size. The liver:body mass ratio was measured for 10 Txnrd1+/+;Gsrnull/nullcontrol and 7 Txnrd1cond/cond;Gsrnull/null;AlbCre1(TR/GR-null liver) mice. Bars show mean±s.e.m. Full size image Figure 2: Survival and physiological characteristics of mice with TR/GR-null livers. ( a – f ) Histopathology. As indicated at left, control GR-null livers ( a , b ) or AlbCre-driven TR/GR-null livers ( c – f ) are shown from P22 ( a – e ) or P56 ( f ) mice. Higher magnification images show representative centrolobular ( a , c ) or periportal ( b , d ) regions. White arrow, tract of apparent oval cells; yellow arrows, leukocytic foci; green arrow, necrotic focus, black arrow, biliary expansion. C, central veins; P, portal triad. Scale bars, 100 μm on all panels. ( g ) Survival of mice with AlbCre-driven TR/GR-null livers. Fifty-one pups from 20 litters with AlbCre-driven TR/GR-null livers were followed. No mice were lost before P32. Between P32 and P42, 15% of the mice were lost. Only one additional loss occurred thereafter (at P55). ( h ) Gender-specific fecundity. Genotypes of sires and dams for each of four mating classes, as well as the number of litters produced and the pups weaned, are indicated at bottom. For a control (first bar from left), production for the TR-null liver colony was monitored over 13 litters (73 pups), giving an average of 5.6 pups/litter. Fecundity was similar in the mice in which Alb ICE drives conversion of livers to TR/GR-null (4.6 pups/litter, second bar from left). Fecundity was also similar in matings where the sires had AlbCre-driven TR/GR-null livers and the dams had GR-null livers (third bar from left, 5.5 pups/litter). However, when dams with TR/GR-null livers were mated with sires with GR-null livers, production was only 70% (fourth bar from left, 3.9 pups/liter), which was significantly less than the controls (*, P <0.01). None of the first three conditions differed significantly from each other. The five oldest production breeders with TR/GR-null livers in the colony, as of this writing, are all over 365 days old (two female and three male) and in combination have weaned ~30 litters. ( i ) Adult (P49–64) TR/GR-null liver size. The liver:body mass ratio was measured for 10 Txnrd1 +/+ ;Gsr null/null control and 7 Txnrd1 cond/cond ;Gsr null/null ;AlbCre 1 (TR/GR-null liver) mice. Bars show mean±s.e.m. 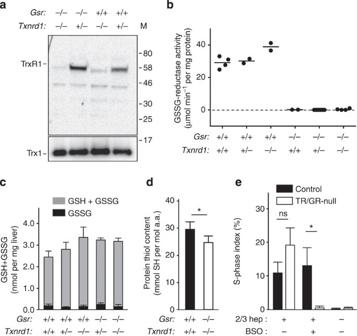Figure 3: Redox homeostasis in TR/GR-null livers. (a) Immunoblots for TrxR1 (top) or Trx1 (below). Hepatocytic genotypes at Gsr and Txnrd1 loci are indicated. M, molecular size markers (kDa). (b) NADPH-dependent GSSG-reductase activity. Hepatocytic genotypes at the Gsr and Txnrd1 loci are indicated; each dot represents one animal. (c) Hepatic levels of total glutathione (GSH+GSSG) and oxidized glutathione disulfide (GSSG) are shown.n=4 animals each for wild-type and TR/GR-null livers (first and last bars), and two to seven animals each for other genotypes; bars represent mean±s.e.m. No differences in GSH+GSSG levels were significant, Student’st-test. Mean GSSG values were, from left to right, 0.17, 0.09, 0.15, 0.32 and 0.12 nmol mg−1liver, respectively. (d) Total protein thiol content in wild-type and TR/GR-null livers. Acid-precipitated total liver proteins were resuspended in acidic denaturing buffer and reacted with 4,4′-dithiol dipyridine. Comparison with a standard curve was used to quantify protein thiol (SH) content and this was normalized to total amino acid (a.a.) content.n=9 wild-type and 8 TR/GR-null livers. (e) Proliferation rates in regenerating or resting livers. Mice were either 2/3 hepatectomized or not. As indicated, BSO was administered 32 h later and 2 h after that bromodeoxyuridine (BrdU) was administered. Livers were harvested 12 h later and BrdU-labelled (S phase) nuclei were enumerated.n=3–5 for each condition; graphs show mean and s.e.m. *P≤0.05, Student’st-test. Full size image Figure 3: Redox homeostasis in TR/GR-null livers. ( a ) Immunoblots for TrxR1 (top) or Trx1 (below). Hepatocytic genotypes at Gsr and Txnrd1 loci are indicated. M, molecular size markers (kDa). ( b ) NADPH-dependent GSSG-reductase activity. Hepatocytic genotypes at the Gsr and Txnrd1 loci are indicated; each dot represents one animal. ( c ) Hepatic levels of total glutathione (GSH+GSSG) and oxidized glutathione disulfide (GSSG) are shown. n =4 animals each for wild-type and TR/GR-null livers (first and last bars), and two to seven animals each for other genotypes; bars represent mean±s.e.m. No differences in GSH+GSSG levels were significant, Student’s t -test. Mean GSSG values were, from left to right, 0.17, 0.09, 0.15, 0.32 and 0.12 nmol mg −1 liver, respectively. ( d ) Total protein thiol content in wild-type and TR/GR-null livers. Acid-precipitated total liver proteins were resuspended in acidic denaturing buffer and reacted with 4,4′-dithiol dipyridine. Comparison with a standard curve was used to quantify protein thiol (SH) content and this was normalized to total amino acid (a.a.) content. n =9 wild-type and 8 TR/GR-null livers. ( e ) Proliferation rates in regenerating or resting livers. Mice were either 2/3 hepatectomized or not. As indicated, BSO was administered 32 h later and 2 h after that bromodeoxyuridine (BrdU) was administered. Livers were harvested 12 h later and BrdU-labelled (S phase) nuclei were enumerated. n =3–5 for each condition; graphs show mean and s.e.m. * P ≤0.05, Student’s t -test. Full size image Methionine is the precursor of cysteine in TR/GR-null livers As TR/GR-null hepatocytes required GSH synthesis for DNA replication but could not reduce GSSG, we inferred that cytosolic disulfide-reducing power came from de novo synthesis of GSH used in single-turnover reactions. With no ability to reductively recycle GSSG back into GSH, the TR/GR-null hepatocytes would need to excrete the GSSG, which was indeed the case (see below). However, it remained unclear how the hepatocytes would obtain the cysteine precursor required for GSH production. The oxidizing environment of blood plasma rapidly oxidizes cysteine, which is therefore typically transported into cells as its disulfide form, cystine [11] . Subsequently, cystine needs to be reduced intracellularly by the Trx- or the GSH-system to yield cysteine [8] , [11] ; however, both of these systems are disrupted in TR/GR-null hepatocytes. By contrast, the methionine cycle and trans -sulfuration pathway, in combination (MTS), can convert the essential amino acid methionine into cysteine without a disulfide reduction reaction [24] , [25] . To test whether the MTS pathway was supporting the TR/GR-null livers, we treated mice with single-dose challenges by inhibitors of cystine uptake (sulfasalazine, SSZ), possible cysteine uptake (2-aminobicyclo-(2,2,1)-heptane-2-carboxylic acid, BCH), conversion of methionine into cysteine by MTS (propargylglycine, PPGG, which inhibits trans -sulfuration and not the methionine cycle), or synthesis of GSH (BSO) [11] . Although neither SSZ nor BCH affected mice with TR/GR-null livers ( Fig. 4a,b , red lines), a single dose of either PPGG or BSO caused rapid deterioration of these mice ( Fig. 4c,d , red lines). None of the inhibitors affected control mice having an active allele of Txnrd1 ( Fig. 4a–d , black lines). This revealed that both MTS-based cysteine synthesis and de novo GSH synthesis were continuously required to complement the TR/GR-null hepatocytes. Histological analyses revealed that BSO or PPGG treatment induced global necrosis of TR/GR-null livers ( Fig. 4e–g ). 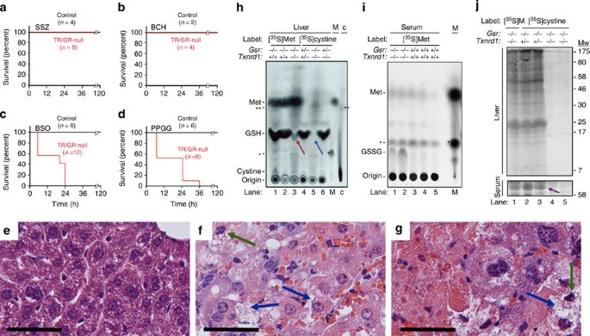Figure 4: TR/GR-null livers requiretrans-sulfuration. (a–d) Adult mice with TR/GR-null livers (genotype Txnrd1cond/cond;Gsr−/−;AlbCre1; red lines) or controls with one active Txnrd1 allele (genotype Txnrd1cond/+;Gsr−/−;AlbCre1; black lines) were treated at time zero with a single dose of SSZ, BCH, BSO or PPGG, as indicated. (e–g) Haematoxylin and eosin-stained histology of TR/GR-null livers following no treatment (e), treatment with BSO (f), or treatment with PPGG (g). Blue arrows, necrotic hepatocytes; green arrows, pyknotic nuclei. Scale bars 50 μm. (h) TLC of [35S]-labelled metabolites from livers 90 min after [35S]methionine (Met) (lanes 1–3) or [35S]cystine (lanes 4–6) administration. Lane M, trace of the [35S]Met labelling mix. Asterisk, spontaneous decay product of [35S]Met that migrated slower than GSH but faster than GSSG. Lane c, trace of [35S]cystine labelling mix verifying that most of the label is cystine; little is in the faster-migrating cysteine form (Cys) (double asterisk). Migration positions of Met, Cys, GSH, GSSG and cystine standards are indicated at the left. (i) TLC analysis of [35S]-labelled serum metabolites 45 min after [35S]Met administration. Asterisks as inh. (j) SDS–PAGE of [35S]-labelled proteins from the liver (top) or serum (below) 45 min after [35S]Met (lane 1) or [35S]cystine (lanes 2–5) administration. Mw, molecular-weight markers. Purple arrow, serum albumin. Figure 4: TR/GR-null livers require trans -sulfuration. ( a – d ) Adult mice with TR/GR-null livers (genotype Txnrd1 cond/cond ;Gsr −/− ;AlbCre 1 ; red lines) or controls with one active Txnrd1 allele (genotype Txnrd1 cond/+ ;Gsr −/− ;Alb Cre1 ; black lines) were treated at time zero with a single dose of SSZ, BCH, BSO or PPGG, as indicated. ( e – g ) Haematoxylin and eosin-stained histology of TR/GR-null livers following no treatment ( e ), treatment with BSO ( f ), or treatment with PPGG ( g ). Blue arrows, necrotic hepatocytes; green arrows, pyknotic nuclei. Scale bars 50 μm. ( h ) TLC of [ 35 S]-labelled metabolites from livers 90 min after [ 35 S]methionine (Met) (lanes 1–3) or [ 35 S]cystine (lanes 4–6) administration. Lane M, trace of the [ 35 S]Met labelling mix. Asterisk, spontaneous decay product of [ 35 S]Met that migrated slower than GSH but faster than GSSG. Lane c, trace of [ 35 S]cystine labelling mix verifying that most of the label is cystine; little is in the faster-migrating cysteine form (Cys) (double asterisk). Migration positions of Met, Cys, GSH, GSSG and cystine standards are indicated at the left. ( i ) TLC analysis of [ 35 S]-labelled serum metabolites 45 min after [ 35 S]Met administration. Asterisks as in h . ( j ) SDS–PAGE of [ 35 S]-labelled proteins from the liver (top) or serum (below) 45 min after [ 35 S]Met (lane 1) or [ 35 S]cystine (lanes 2–5) administration. Mw, molecular-weight markers. Purple arrow, serum albumin. Full size image Next we performed metabolic radiolabelling experiments with either [ 35 S]methionine or [ 35 S]cystine. Using either amino acid, a metabolite was radiolabelled in control livers that migrated as GSH in thin layer chromatography (TLC) ( Fig. 4h ). In TR/GR-null livers [ 35 S]methionine labelled this metabolite (red arrow), however [ 35 S]cystine did not (blue arrow). Following [ 35 S]methionine labelling, serum metabolites from mice with TR/GR-null livers showed a labelled species that migrated as GSSG in TLC, which was much less abundant in serum of control mice ( Fig. 4i ). These results suggested the TR/GR-null livers metabolized [ 35 S] from exogenously supplied [ 35 S]methionine, via cysteine and GSH, to GSSG, which was then excreted. The results also confirmed that exogenously supplied [ 35 S]cystine was not effectively used for GSH synthesis in TR/GR-null livers. Both methionine and cysteine are required for protein synthesis. After inoculation with either [ 35 S]methionine or [ 35 S]cystine, proteins became radiolabelled in control livers; however, only [ 35 S]methionine gave substantial radiolabelling of proteins in TR/GR-null livers ( Fig. 4j ). In serum, albumin, which is synthesized by hepatocytes and contains 36 cysteine and 7 methionine residues, was radiolabelled by either [ 35 S]methionine or [ 35 S]cystine in control animals, but was only substantially radiolabelled by [ 35 S]methionine in mice having TR/GR-null livers ( Fig. 4j , bottom, purple arrow). These results showed that cystine cannot be effectively used as a cysteine precursor in TR/GR-null livers. The use of intracellular NADPH by TrxR or GR to drive cytosolic thiol–disulfide exchange reactions in a reducing direction is considered a nearly universal property of living systems. Here we show that mice lacking all GR activity and constitutively also lacking hepatocytic TrxR1 can nonetheless maintain sufficient hepatic redox homeostasis and intermediary metabolism for long-term survival. Moreover, our data exclude the possibility that alternative NADPH-dependent oxidoreductases make substantial contributions to supporting disulfide reduction reactions in the TR/GR-null livers. For example, in addition to TrxR1, cells contain the mitochondrial TrxR2 enzyme [17] . Previously, we have shown that no alternative sources of TrxR activity, including TrxR2, support DNA replication in GSH-depleted TrxR1-null livers [10] . Consistent with this, TR/GR-null livers are metabolically addicted to MTS-driven synthesis of cysteine and de novo synthesis of GSH ( Figs 3e and 4c,d ), highlighting a critical role of GSH in survival of the TR/GR-null livers. The absence of NADPH-dependent GSSG reduction activity ( Fig. 3b ) and negligible utilization of exogenous cystine by TR/GR-null livers ( Fig. 4h,j ) further suggest the TR/GR-null hepatocytes lack activities that could, via disulfide reduction, generate substantial levels of cysteine as a source of disulfide-reducing power or for protein synthesis. Whereas other NADPH-dependent oxidoreductases expressed in the livers lacking TrxR1, such as carbonyl reductases or NADPH–quinone dehydrogenase [20] , [23] , might contribute to redox homeostasis in the TR/GR-null livers by reducing non-sulfur substrates, our results suggest that disulfide-reducing activities in TR/GR-null livers are not markedly supported by processes other than de novo GSH synthesis. Normal liver exhibits substantial MTS activity, which uses dietary methionine to generate S- adenosylmethionine, recycle 5-methyltetrahydrofolate to tetrahydrofolate and produce substantial amounts of cysteine, the latter of which can be used for de novo GSH synthesis and protein synthesis [11] , [24] , [26] ( Fig. 5a ). In TR/GR-null livers, as the intracellular transfer of reducing power via NADPH and GR or TrxR1 was ablated, extracellular methionine became the sole source of cysteine for both GSH as well as protein synthesis, and thus the sole source of sulfur-containing molecules. Moreover, methionine, via cysteine and GSH, thereby became the sole detectable source of cytosolic disulfide-reducing power in TR/GR-null livers ( Fig. 5b ). 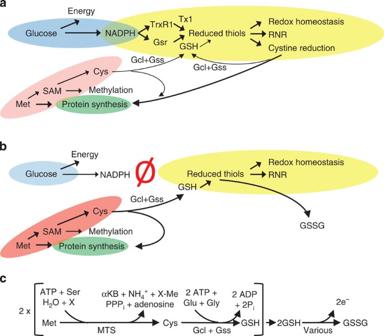Figure 5: Alternative pathways can maintain redox homeostasis in hepatocytes. (a) In normal hepatocytes, glucose utilization by the pentose phosphate pathway (blue) yields NADPH, which feeds the GSH and Trx1 systems (yellow). These systems maintain cytosolic redox homeostasis, drive ribonucleotide reductase (RNR) and reduceL-cystine into cysteine. MTS (red) supplies SAM for methylation reactions and provides an alternative source of cytosolic cysteine, which is used for protein- (green) and GSH-synthesis. (b) Concomitant genetic ablation of GR and TrxR1 (red ‘Ø’) in TR/GR-null livers uncouples glucose oxidation and NADPH from the major disulfide reduction systems. In this case, MTS uses dietary methionine to provide an alternative source of cytosolic cysteine. This cysteine is sufficient to support protein synthesis and to serve as the sole source of cytosolic disulfide reduction power in TR/GR-null livers without the use of NADPH. (c) Balanced reaction for utilization of two electrons of reducing power in TR/GR-null hepatocytes. Gcl, glutamate-cysteine ligase; Gss, GSH-synthase; PPPi, inorganic triphosphate; X, any methyl- (Me-) acceptor for SAM-dependent methyl transferase activity. Figure 5: Alternative pathways can maintain redox homeostasis in hepatocytes. ( a ) In normal hepatocytes, glucose utilization by the pentose phosphate pathway (blue) yields NADPH, which feeds the GSH and Trx1 systems (yellow). These systems maintain cytosolic redox homeostasis, drive ribonucleotide reductase (RNR) and reduce L -cystine into cysteine. MTS (red) supplies SAM for methylation reactions and provides an alternative source of cytosolic cysteine, which is used for protein- (green) and GSH-synthesis. ( b ) Concomitant genetic ablation of GR and TrxR1 (red ‘Ø’) in TR/GR-null livers uncouples glucose oxidation and NADPH from the major disulfide reduction systems. In this case, MTS uses dietary methionine to provide an alternative source of cytosolic cysteine. This cysteine is sufficient to support protein synthesis and to serve as the sole source of cytosolic disulfide reduction power in TR/GR-null livers without the use of NADPH. ( c ) Balanced reaction for utilization of two electrons of reducing power in TR/GR-null hepatocytes. Gcl, glutamate-cysteine ligase; Gss, GSH-synthase; PPPi, inorganic triphosphate; X, any methyl- (Me-) acceptor for SAM-dependent methyl transferase activity. Full size image Control and TR/GR-null livers had similar steady-state levels of GSH ( Fig. 3c ), yet 90 min after metabolic labelling with [ 35 S]methionine the TR/GR-null livers contained substantially less [ 35 S] in hepatic GSH pools ( Fig. 4h , red arrow). As the TR/GR-null livers were unable to incorporate [ 35 S] from cystine into GSH ( Fig. 4h , blue arrow), we suspect that the relatively low specific activity of the hepatic GSH pool stemmed from a high rate of GSH turnover in these livers. This interpretation is consistent with the appearance of increased levels of [ 35 S]-labelled GSSG in the serum of animals with TR/GR-null livers following metabolic labelling with [ 35 S]methionine ( Fig. 4i ). Quantitative metabolite flux analyses will be required to better understand how the demands for de novo cysteine and GSH biosynthesis in the TR/GR-null livers have an impact on the transit of amino acids through competing pathways. The long-term survival of mice with TR/GR-null livers indicates that homeostasis, that is, a sustainable physiological function, is achieved in the hepatocytes as well as in all organs of these mice. Although steady-state levels and redox status of GSH is near-normal ( Fig. 3c ), total protein thiol content is lower in the TR/GR-null as compared with wild-type livers ( Fig. 3d ), suggesting the redox equilibrium in these livers is more oxidizing. The diminished protein thiol content, susceptibility to perturbations in methionine metabolism, evidence of chronic low-grade hepatic pathology and occasional spontaneous death in mice with TR/GR-null livers suggest that homeostasis in these animals is at the ‘brink of failure’. Future studies on these mice will probably lead to a better understanding of actual hepatocyte redox requirements, especially under conditions of increased oxidative burden. GR-dependent recycling of GSSG oxidizes one molecule of NADPH and yields two molecules of GSH. By comparison, conversion of methionine to cysteine via MTS hydrolyses three ATP-phosphodiester bonds and consumes one molecule of serine to produce one molecule of cysteine, one molecule of α-ketobutyrate and one molecule of adenosine [27] . Subsequently, GSH synthesis using this cysteine precursor hydrolyses two more ATP–phosphodiester bonds and consumes one glutamate and one glycine [11] . Thus, in the TR/GR-null livers, cells must use at least ten ATP–phosphodiester bonds and two molecules each of methionine, glutamate, glycine and serine to acquire two molecules of GSH ( Fig. 5c ). All four amino acids used in this process are readily salvaged from plasma. In addition, the energy used as ATP in this process is probably conserved by mitochondrial conversion of α-ketobutyrate to succinyl-CoA followed by complete oxidation to four CO 2 through two transits of the citric acid cycle and generation of ATP by oxidative phosphorylation ( Fig. 6 ). Thereby, utilization of methionine for obtaining reducing power might, surprisingly, be energetically more favourable than the reductive recycling of GSSG by GR. However, the altered flux of amino acids and their metabolites through transporters, cytosolic pools, MTS and competing pathways when using methionine as the sole source of reducing power might still be more taxing to the cells. 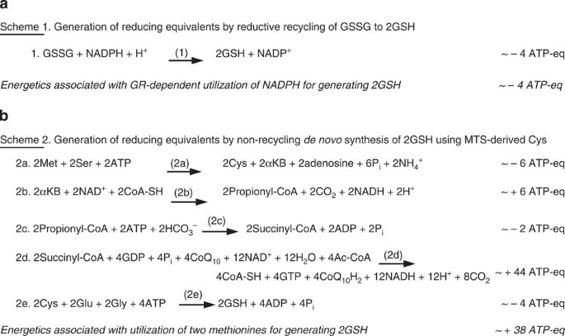Figure 6: Relative energetics of using intracellular NADPH versus dietary amino acids for reducing power. Schematics are presented for general comparison of the bioenergetics of the alternative sources of GSH discussed in this study, initiating with either NADPH+GSSG in Scheme 1 or with Met+Ser+Glu+Gly in Scheme 2. The energy gain from NADPH production in the PPP is not considered, as this is only one of several catabolic pathways for glucose. In addition, no energetic consumption was estimated for acquisition of Met, Ser, Glu, or Gly in reactions 2A or 2E, because these amino acids are readily salvaged from plasma. (a) Scheme 1. Generation of reducing equivalents by reductive recycling of GSSG to 2GSH. (b) Scheme 2. Generation of reducing equivalents by non-recyclingde novosynthesis of GSH using Cys synthesizedde novofrom Met. Pathways/enzymes: (1) GR; (2a) MTS; (2b) branched chain α-ketoacid dehydrogenase complex; (2c) propionyl-CoA carboxylase, methylmalonyl-CoA racemase and methylmalonyl-CoA mutase; (2d) citric acid cycle; (2e) Gcl and Gss. Reactions 1, 2a and 2e are cytosolic; 2b, 2c and 2d are mitochondrial. Energetic values are given as ATP-equivalents (ATP-eq) and based on estimates of 1 NADPH=4 ATP; 1 NADH=3 ATP; 1 CoQ10H2=2 ATP; 1 GTP=1 ATP. Although utilization of two Met to obtain two electrons of reducing potential consumes ten ATP-phosphodiester bonds in the primary reactions (2a and 2e), the potential energy yield from mitochondrial utilization of 2 α-ketobutyrate, a byproduct of reaction 2a, would make this pathway energetically favourable, with a potential net gain of ~38 ATP-eq for generating two GSH as compared with a loss of ~4 ATP-eq for GR-catalysed reductive recycling of GSSG to 2 GSH. Figure 6: Relative energetics of using intracellular NADPH versus dietary amino acids for reducing power. Schematics are presented for general comparison of the bioenergetics of the alternative sources of GSH discussed in this study, initiating with either NADPH+GSSG in Scheme 1 or with Met+Ser+Glu+Gly in Scheme 2. The energy gain from NADPH production in the PPP is not considered, as this is only one of several catabolic pathways for glucose. In addition, no energetic consumption was estimated for acquisition of Met, Ser, Glu, or Gly in reactions 2A or 2E, because these amino acids are readily salvaged from plasma. ( a ) Scheme 1. Generation of reducing equivalents by reductive recycling of GSSG to 2GSH. ( b ) Scheme 2. Generation of reducing equivalents by non-recycling de novo synthesis of GSH using Cys synthesized de novo from Met. Pathways/enzymes: (1) GR; (2a) MTS; (2b) branched chain α-ketoacid dehydrogenase complex; (2c) propionyl-CoA carboxylase, methylmalonyl-CoA racemase and methylmalonyl-CoA mutase; (2d) citric acid cycle; (2e) Gcl and Gss. Reactions 1, 2a and 2e are cytosolic; 2b, 2c and 2d are mitochondrial. Energetic values are given as ATP-equivalents (ATP-eq) and based on estimates of 1 NADPH=4 ATP; 1 NADH=3 ATP; 1 CoQ10H2=2 ATP; 1 GTP=1 ATP. Although utilization of two Met to obtain two electrons of reducing potential consumes ten ATP-phosphodiester bonds in the primary reactions (2a and 2e), the potential energy yield from mitochondrial utilization of 2 α-ketobutyrate, a byproduct of reaction 2a, would make this pathway energetically favourable, with a potential net gain of ~38 ATP-eq for generating two GSH as compared with a loss of ~4 ATP-eq for GR-catalysed reductive recycling of GSSG to 2 GSH. Full size image The liver regulates systemic homeostasis of sugars, lipids, amino acids, nucleosides, vitamins, steroid hormones and other compounds [28] , including sulfur- and seleno-amino acids [29] , with hepatocyte Trx1 and GSH systems participating in these processes [11] , [30] . Here, however, we report that hepatic function and, thereby, organismal survival, is sustained in mice lacking both TrxR1 and GR in all hepatocytes. Dietary methionine is shown to be an adequate source of sulfur amino acids and disulfide reduction power. This reveals how essential cytosolic disulfide reduction systems, at least in liver, can remain functional without using NADPH, illustrating the robustness of redox homeostasis and identifying methionine as an alternative fuel for redox processes. Animals This study adhered to the United States National Institutes of Health and United States Department of Agriculture guidelines for care and use of animals in research. All animal protocols were reviewed and approved by the Montana State University Institutional Animal Care and Use Committee. The alleles used in this study have been published elsewhere, as described in the text. Except where indicated otherwise, all analyses shown were done on mice of either gender between 8 and 12 weeks of age. Mice were genotyped by PCR using tail biopsies harvested between P10 and P14. Mice were kept under specialized care conditions, including continuous-flow HEPA-filtered air cages (Tecniplast), sterilized bedding and enrichment, free access to sterilized feed (Picolabs 5058) and sterilized water, and on a 14:10 light:dark cycle. For hydrodynamic delivery of Cre to liver hepatocytes, mice received a single tail-vein injection of lactated Ringer’s solution equal to 10% of their body weight, containing 5 μg of plasmid pCMVpCreSVtx [31] . For Tamoxifen-induced conversion of all hepatocytes in mice, ROSA mT-mG/mT-mG ; Txnrd1 cond/cond ; Gsr null/null ; Alb ICE/+ mice, having an allele of the Alb ICE (for Alb-IRES-CreERT2) knock-in allele [32] (a generous gift from P. Chambon and D. Metzger, Illkirch, France), in which an IRES (internal ribosomal entry site)- driven second cistron targeted into the 3′ untranslated region of the endogenous Alb locus was used to provide strong hepatocyte-specific transcription and translation of the Tamoxifen-inducible CreERT2 protein. Adult mice were administered a single intraperitoneal (i.p.) dose of 0.5 ml vegetable oil containing 0.5 mg ml −1 4-OH-Tamoxifen and 1.5 mg ml −1 Tamoxifen-free base, which resulted in complete conversion of all hepatocytes to green. No feed or water supplements were used for the data presented. To assess survival, pups from 20 litters with different parental combinations were followed. Based on Mendelian segregation of alleles, we expected these litters to yield a total of 41 pups with allelic combinations that would generate AlbCre-driven TR/GR-null livers. Genotype analyses performed on tail biopsies taken at P10–P14 (dark triangle) indicated that 51 pups had TR/GR-null livers. This value did not differ significantly from expected ( T -test, P =0.295), suggesting that zygotes having an allelic combination that should yield TR/GR-null livers survived equivalently to their littermates. At tail biopsy, each animal was given a unique identifier and the 51 mice with TR/GR-null livers were followed with daily monitoring thereafter. Losses include all mice that were either found dead or humanely killed on becoming moribund. Statistics Except as indicated, all analyses were repeated at least in triplicate and representative data are presented. Where applicable, the number ( n ) is given in figures or legends. Quantitative data is presented as averages±s.e.m. Significance was tested on pairwise analyses using a Student’s t -test with P ≤0.05 indicating significance. Surgeries and S-phase indexes Partial (2/3) hepatectomies were performed aseptically under isofluroane anaesthesia. The median and left lateral lobes were ligated and resected, incisions were sutured and surface-exposed sutures were secured with VetBond (3 M) tissue adhesive [33] , [34] , [35] . Thirty-six hours after hepatectomy, 5-bromo-2′-deoxyuridine (BrdU, 2.5 μmol in saline, Alfa-Aesar H27260) was injected i.p. Paraffin sections of livers were stained with mouse anti-BrdU-DNA antibody (Sigma-Aldrich, B2531, 1:10) followed by goat-anti-mouse-horseradish peroxidase-conjugated secondary antibody (MP Biomedicals, 55550, 1:3,000). S-phase indexes represent the ratio of BrdU-stained to un-stained hepatocyte nuclei. Analyses were repeated on three to five animals of each condition and >15,000 hepatocyte nuclei were evaluated for each animal [10] , [33] . Inhibitor studies SSZ (MP Biomedicals, 02919944, 5 mg kg −1 ), BCH (Sigma-Aldrich, A7902, 700 mg kg −1 ), PPGG (Sigma-Aldrich, P7888, 0.5 mmol kg −1 ), or BSO (Sigma-Aldrich, B2515, 7.2 mmol kg −1 ) were dissolved in sterile saline and were administered as a single i.p. inoculum in each case [16] , [36] , [37] , [38] , [39] . Redox assays and immunoblotting At the time of killing, the livers were perfused with saline (cardiac portal), excised, cut into ~0.3 g pieces and pieces were either fixed in neutral-buffered formalin for paraffin-embedding and histology or snap-frozen in liquid nitrogen and stored at −80 °C [23] . For immunoblots and GSSG-reductase assays, snap-frozen liver pieces were homogenized in 0.8 ml of ice-cold 50 mM Tris-Cl, pH 7.5, 150 mM NaCl, 2 mM EDTA, 1% Trition X-100, 1 × protease inhibitor (Pierce #88666) [10] , [23] , [33] , [40] . After pelleting debris, protein concentrations of the clarified lysates were determined by Bradford assay (Thermo Scientific, 23238). Liver proteins (25 μg) were boiled in loading buffer containing dithiothreitol (DTT) and SDS, separated on 4%–20% polyacrylamide gradient gels and transferred onto nitrocellulose membranes [10] . After blocking in 5% non-fat milk, membranes were incubated overnight with anti-mouse-TrxR1 or anti-mouse-Trx1 rabbit sera (each used at 1:4,000 dilution, kindly provided by G. Merrill, Oregon State University) followed by goat-anti-rabbit horseradish peroxidase-conjugated secondary antibody and visualization by chemoluminescence (Pierce PicoWest system) [20] . For NADPH-dependent GSSG reduction assays, 50 μg of liver lysate in 10 μl was mixed with 190 μl of reaction mixture containing 1 mM GSSG (Sigma-Aldrich G4626) and 200 μM NADPH (Sigma-Aldrich N7505) in 100 mM potassium phosphate, pH 7.0, 2 mM EDTA [10] , [23] , [41] . Absorbance at 340 nm was followed at 30 °C using a Versamax plate reader (Molecular Devices). A background control lacking GSSG for each sample was subtracted from sample activities. To measure GSH and GSSG levels [10] , [42] , snap-frozen liver pieces (~0.3 g) were homogenized in 0.8 ml of 10 mM HCl and proteins were removed by adding 5-sulfosalicylic acid to 1% (w v −1 ) followed by centrifugation. For GSSG measurements, 2 μl of 2-vinyl pyridine (98%, Sigma-Aldrich 132292) was added to 100 μl of each supernatant and incubated at room temperature for 1 h to alkylate free thiols before reaction. Reaction mixes contained 120 mM NaH 2 PO 4 , pH 7.4, 5.3 mM EDTA, 0.75 mM 5,5′-dithiobis-(2-nitrobenzoic acid (Sigma D8130), 0.24 mM NADPH and 1.2 IU ml −1 GR (Sigma-Aldrich G9297), and either 5 μl (GSH+GSSG assay) or 20 μl (GSSG assay) clarified lysate, and were followed at room temperature by absorbance at 412 nm in a Versamax plate reader. Standard curves prepared in parallel contained GSH or GSSG. Liver GSH and GSSG concentrations were calculated by comparison with standard curves assuming 100% recovery at all steps. Total protein thiol content was determined using 4,4′-dithiodipyridine under denaturing acidic conditions to expose buried cysteines and inhibit ex vivo oxidation [43] , [44] , [45] . Briefly, snap-frozen liver samples were thawed by homogenization in three volumes of ice-cold 10% tricholoroacetic acid. Precipitated macromolecules were collected by centrifugation and were washed three times with 10% trichloroacetic acid. Pellets were dissolved by brief sonication in a volume equivalent to 30 times the starting liver mass of 0.4 M sodium citrate, pH 4.5, 1 mM EDTA, 5% SDS (‘protein samples’). An aliquot of each protein sample (2 μl) was transferred into tubes containing 68 μl 0.1 M sodium citrate, pH 4.5, 1 mM EDTA, 0.3% SDS and 0.5 mM 4,4′-dithiodipyridine (Sigma-Aldrich 143057). Samples were mixed and incubated at room temperature for 30 min. Samples received 130 μl of 0.1 M sodium citrate, pH 4.5, 4 M urea and were incubated another 30 min at room temperature. As a standard curve to calculate thiol content, DTT powder (Gold Biotechnology, DTT50) was freshly dissolved in 0.4 M sodium citrate, pH 4.5, 1 mM EDTA, 5% SDS and a dilution series from 0 to 3 nmol was prepared and assayed in parallel with samples. Absorbance of each sample was read at 324 nm in a Beckman DU 800 spectrophotometer. The molar concentration of free thiols in each liver protein sample was determined by comparison with DTT standard curve, correcting for each molecule of DTT having two thiols. For total protein amino acid content, a separate aliquot of each protein sample (10 μl) was hydrolysed overnight at 95 °C–100 °C in 100 μl of 6 M HCl, dried in a Speed Vac and re-dissolved in 200 μl of 1 × PBS. An aliquot of each (10 μl) was diluted with water to 500 μl and mixed with 500 μl hydrindantin solution, freshly prepared by dissolving 0.1 g ninhydrin (Alpha-Aesar 43846) in 7.3 ml dimethyl sulfoxide, adding 2.5 ml 1.65 M lithium acetate, pH 4.5, and then reducing the ninhydrin by adding 200 μl 0.66 M SnCl2. To generate a standard curve of known amino acid content, a dilution series from 0 to 34 nmol of alanine (FW 89.1 g mol −1 ; Acros 102831000) in 1 × PBS was assayed in parallel with the liver samples. Samples were incubated at 100 °C for 10 min and cooled on ice. Under these conditions, the hydrindantin reacts with the primary amine group on each amino acid, giving a blue colour that was quantified by absorbance at 570 nm [43] . To calculate the number of thiols per total amino acids in the liver samples, the moles of thiols per volume of each protein sample was divided by the moles of amino acids per volume of the same sample. Metabolic labelling [ 35 S]methionine and [ 35 S]cysteine were purchased from MP Biomedicals (MP5100405 and MP5100205, respectively). To generate [ 35 S]cystine, the [ 35 S]cysteine (1 mCi) was incubated with an equal molar amount of fresh hydrogen peroxide overnight at 25 °C, quenched in ten volumes of cystine-free, methionine-free DMEM medium (Sigma-Aldrich, D0422) and stored frozen. Controls on TLC plates showed that nearly all radioactivity migrated as cystine and not as cysteine on these preparations ( Fig. 2h , lane c). For all labelling studies shown, mice were inoculated i.p. with 0.5 ml of methionine-free, cystine-free DMEM containing 0.2 mCi of the indicated labelled amino acid. Animals were killed 45 or 90 min later, as indicated in the text. Blood was collected by clean draw from the inferior vena cava to produce serum; the livers were harvested and snap freezing in liquid nitrogen and stored at −80 °C. Liver fragments were thawed and homogenized by sonication in ~10 volumes of ice-cold buffer containing 50 mM Tris-Cl, pH 7.5, 150 mM NaCl, 2 mM EDTA and 1% Trition X-100 (ref. 23 ). Homogenates were clarified by centrifugation and protein concentrations were determined by Bradford assay. SDS–PAGE protein gels were run with 50 μg of total liver protein or 10 μg of serum protein. Gels were stained with Coomassie, destained, dried and exposed by autoradiography or phosphorimaging. For metabolite analyses, liver homogenates or serum samples were prepared by homogenization in 50% methanol on ice. Samples were incubated overnight at −20 °C and clarified by centrifugation. A portion of the clarified extract was removed to tubes containing five volumes of acetone and proteins were precipitated for 2–20 h at −20 °C. Samples were clarified by centrifugation at 4 °C for 15 min in a microcentrifuge and the clear supernatant was transferred to a new tube. Solvent was removed to completion using a Speed-Vac and the dried metabolite pellet was resuspended in 50% methanol. Samples were spotted onto silica TLC plates (Sigma-Aldrich, Z122785) and were migrated for 16 h using 3:1:1 butanol:acetic acid:water. Metabolites were detected by autoradiography or phosphorimaging. All plates contained non-labelled standards that were visualized after exposure by spraying with ninhydrin staining solution (1 mg ml −1 ninhydrin) in acetone with 0.5% acetic acid and heating at 50 °C until colour developed. Standards used to calibrate TLC were L -methionine (Amresco, E801), L -Cysteine (Sigma-Aldrich, C7755), L -cystine (Chem-Impex International, 00088), L -GSSG (Sigma-Aldrich, G4376) and L -GSH (ICN Biomedicals, 101814). How to cite this article: Eriksson, S. et al. Dietary methionine can sustain cytosolic redox homeostasis in the mouse liver. Nat. Commun. 6:6479 doi: 10.1038/ncomms7479 (2015).